G-CSF supports long-term muscle regeneration in mouse models of muscular dystrophy Duchenne muscular dystrophy (DMD) is a chronic and life-threatening disease that is initially supported by muscle regeneration but eventually shows satellite cell exhaustion and muscular dysfunction. The life-long maintenance of skeletal muscle homoeostasis requires the satellite stem cell pool to be preserved. Asymmetric cell division plays a pivotal role in the maintenance of the satellite cell pool. Here we show that granulocyte colony-stimulating factor receptor (G-CSFR) is asymmetrically expressed in activated satellite cells. G-CSF positively affects the satellite cell population during multiple stages of differentiation in ex vivo cultured fibres. G-CSF could be important in developing an effective therapy for DMD based on its potential to modulate the supply of multiple stages of regenerated myocytes. This study shows that the G-CSF–G-CSFR axis is fundamentally important for long-term muscle regeneration, functional maintenance and lifespan extension in mouse models of DMD with varying severities. Adult skeletal muscle has its own stem cell population known as satellite cells (SCs). After muscle injury, quiescent SCs are activated and then proliferate and differentiate into mature skeletal muscle to ensure that muscle function is recovered. SCs are at the top of the hierarchy of differentiating stages in adult myocytes, followed by myoblasts, immature myocytes and matured myocytes. Thus, maintaining the homoeostasis of skeletal muscle function over the long term requires a well-preserved population of SCs. However, SCs are still heterogenic, and among the distinct differentiation stages, the satellite stem cell population must be maintained to preserve their stemness, that is, long-term self-renewal and differentiation abilities. Accumulating data indicate that SCs maintain their population by asymmetric cell division [1] , [2] , [3] , [4] . The different differentiation stages of SCs are distinguishable by the expression of specific markers such as PAX7 and MYOD; PAX7+/MYOD− cells are quiescent, PAX7+/MYOD+ cells are activated and PAX7−/MYOD+ cells are differentiating. Interestingly, some activated SCs exhibit asymmetric MYOD distribution within the cells, and each daughter cell is either PAX7+/MYOD+ or PAX7+/MYOD−, the latter of which retains the quiescent state [5] . Such evidence indicated that asymmetric protein distribution produces asymmetric cell division, which has a critical role in maintaining the SC population. In our previous screen for myocyte differentiation-promoting factors [6] , [7] , we noted markedly elevated expression of granulocyte colony-stimulating factor receptor (G-CSFR, encoded by csf3r ) in the developing somite [8] . Furthermore, G-CSFR was transiently expressed in regenerating myocytes of adult injured skeletal muscle, and extrinsic G-CSF supported short-term muscle regeneration in cardiotoxin-induced skeletal muscle injury [9] and crush injury [10] . However, although we found high G-CSFR expression in regenerating immature myocytes, whether G-CSFR would be expressed in SCs and whether G-CSF signalling would affect the SC population in skeletal muscle remain unclear. Duchenne muscular dystrophy (DMD) is one of the most common inheritable muscle diseases in humans [11] , [12] . It is an X-linked progressive disease that affects approximately one in 3,500 male live births [13] . DMD is caused by a mutation in the gene encoding dystrophin , which links the internal muscle cytoskeleton to the extracellular matrix, enabling the lateral transmission of force from within muscle cells to the surrounding matrix. Mutations in the dystrophin gene lead to dystrophin deficiency at the myofibre membrane and progressive muscle fibre degeneration [14] , [15] . The absence of dystrophin increases the fragility of the sarcolemma, which is susceptible to even mild stress [16] . Subsequent injury results in myofibre necrosis, followed by repetitive degeneration and regeneration supported by innate SCs. In DMD, muscle regeneration initially supports the mutation-driven functional impairment; however, such regeneration is eventually attenuated due to stem cell exhaustion [17] . Therapy that induces effective long-term skeletal muscle regeneration is, therefore, crucially needed for DMD. Long-term muscle regenerative therapy for conditions such as DMD relies on increasing the pool of functional myocytes and maintaining the pool of SCs. We showed that G-CSFR is asymmetrically distributed in activated SCs, and that G-CSF increases the population of SCs via the G-CSF–G-CSFR axis in ex vivo cultured myofibres. On the basis of this, we hypothesized that G-CSF could be important in developing an effective therapy for DMD based on its potential to modulate the supply of multiple stages of regenerated myocytes. It is surprising that haploinsufficiency of G-CSFR leads to early lethality in DMD model mice, indicating that dose reduction of the G-CSF/G-CSFR system could not support the balance between degeneration and regeneration. We also showed that G-CSF administration in mice with severe DMD markedly improves the phenotype, including muscle pathology, functioning and lifespan. Together, our data suggested that the G-CSF–G-CSFR axis is fundamentally important for long-term muscle regeneration, functional maintenance and lifespan extension in DMD mouse models with varying severities. G-CSFR is expressed in activated SCs To explore the precise expression pattern of G-CSFR in skeletal muscle, we examined the SCs on isolated myofibres from the extensor digitorum longus (EDL) muscles of wild-type mice. This model preserves the physiological behaviour of SCs through activation, proliferation and differentiation on myofibres. In the isolated myofibres, PAX7+ quiescent SCs showed no G-CSFR expression by immunostaining at the time of myofibre isolation ( Fig. 1a ). G-CSFR expression was observed in the PAX7+ cells after 6 h ( Fig. 1a,c ), when MYOD expression also appeared ( Fig. 1b ; Supplementary Fig. 1a ). G-CSFR expression was still apparent at 48 h in the MYOGENIN+ SCs, which are committed to differentiation ( Supplementary Fig. 1b,c ) [18] . By 24 and 48 h, the number of G-CSFR-expressing cells increased to ∼ 94% of PAX7+ cells ( Fig. 1c ). 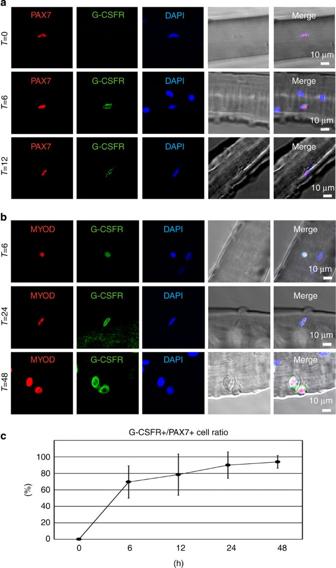Figure 1: G-CSFR is expressed in activated satellite cells. (a) Immunostaining of satellite cells on myofibres isolated from EDL muscles for PAX7 (red) and G-CSFR (green), including nuclei stained with DAPI (blue) and bright-field images, at 0 h (T=0), 6 h (T=6) and 12 h (T=12). Scale bar, 10 μm. (b) Immunostaining of satellite cells on myofibres for MYOD (red) and G-CSFR (green) at 6 h (T=6), 24 h (T=24) and 48 h (T=48). Scale bar, 10 μm. (c) The G-CSFR+/PAX7+ cell ratio at 0, 6, 12, 24 and 48 h (T=0:n=53;T=6:n=73;T=12:n=45;T=24:n=41;T=48:n=297; each myofibre:n=20–30). All myofibres were obtained from∼10-week-old wild-type mice. Data are shown as mean±s.d. DAPI, 4',6-diamidino-2-phenylindole dihydrochloride. Figure 1: G-CSFR is expressed in activated satellite cells. ( a ) Immunostaining of satellite cells on myofibres isolated from EDL muscles for PAX7 (red) and G-CSFR (green), including nuclei stained with DAPI (blue) and bright-field images, at 0 h ( T =0), 6 h ( T =6) and 12 h ( T =12). Scale bar, 10 μm. ( b ) Immunostaining of satellite cells on myofibres for MYOD (red) and G-CSFR (green) at 6 h ( T =6), 24 h ( T =24) and 48 h ( T =48). Scale bar, 10 μm. ( c ) The G-CSFR+/PAX7+ cell ratio at 0, 6, 12, 24 and 48 h ( T =0: n =53; T =6: n =73; T =12: n =45; T =24: n =41; T =48: n =297; each myofibre: n =20–30). All myofibres were obtained from ∼ 10-week-old wild-type mice. Data are shown as mean±s.d. DAPI, 4',6-diamidino-2-phenylindole dihydrochloride. Full size image Asymmetrically expressed G-CSFR in activated SCs Unexpectedly, we found that G-CSFR is asymmetrically distributed within migrating SCs obtained from isolated myofibres at day 5 ( Fig. 2a ). This asymmetric distribution of G-CSFR was apparent in ∼ 20% of PAX7+ SCs at 72 h ( Fig. 2b ). Syndecan-4 (SDC4) was expressed in the activated SCs until mature myocyte fusion occurred; thus, paired SDC4+ cells were characterized as the daughter cells of SC division [19] , [20] . The majority of paired SDC4+ cells showed equivalent expression of G-CSFR (94.4%; Fig. 2c ), but in the remaining 5.6% of paired SDC4+ cells, G-CSFR was detectable in only one daughter cell ( Fig. 2d ). Similarly, single SDC4+ SCs either express G-CSFR or not ( Fig. 2e,f ). In ∼ 5% of paired PAX7+/SDC4+ cells, one daughter cell highly expressed G-CSFR; in the other daughter cell, G-CSFR expression was not observed ( Fig. 2g ). In addition, in ∼ 5% of paired PAX7+ cells, one G-CSFR+ daughter cell highly expressed MYOD, whereas no MYOD expression observed in the other ( Fig. 2h ). These data suggested that G-CSFR is expressed from the activation of SCs through asymmetrical distribution during the first divisions but is not expressed in the self-renewing PAX7+/MYOD− SCs ( Supplementary Fig. 2 ). 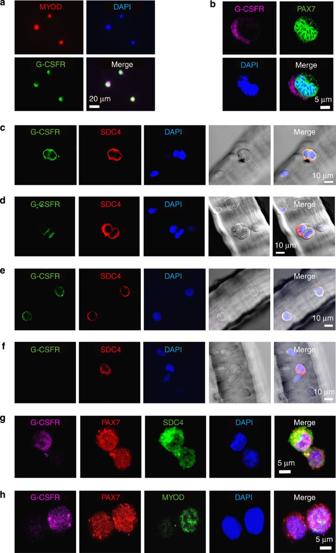Figure 2: G-CSFR is asymmetrically expressed in activated satellite cells. (a) Immunostaining of satellite cells for MYOD (red), G-CSFR (green) and DAPI (blue) at day 5. Scale bar, 20 μm. (b) Immunostaining of satellite cells for G-CSFR (purple), PAX7 (green) and DAPI (blue) at day 3. Scale bar, 5 μm. (c) Immunostaining of dividing satellite cells on myofibres for G-CSFR (green), SDC4 (red) and DAPI (blue), as well as bright-field (BF) images, at 48 h (satellite cells with symmetric G-CSFR expression:n=51; satellite cells with asymmetric expression:n=3). Scale bar, 10 μm. (d) Immunostaining of dividing satellite cells on myofibres for G-CSFR (green), SDC4 (red) and DAPI (blue), as well as BF images, at 48 h. Scale bar, 10 μm. (e,f) Immunostaining of satellite cells on myofibres for SDC4 (red), G-CSFR (green) and DAPI (blue), as well as BF images, at 48 h. Scale bar, 10 μm. (g) Immunostaining of cultured dividing satellite cells for G-CSFR (purple), PAX7 (red), SDC4 (green) and DAPI (blue). Scale bar, 5 μm. (h) Immunostaining of cultured dividing satellite cells for G-CSFR (purple), PAX7 (red), MYOD (green) and DAPI (blue) at day 3 (among 273 dividing satellite cells, dividing satellite cells with symmetric G-CSFR expression:n=5; dividing satellite cells with asymmetric expression:n=268). Scale bar, 5 μm. All myofibres were obtained from∼10-week-old wild-type mice. DAPI, 4',6-diamidino-2-phenylindole dihydrochloride. Figure 2: G-CSFR is asymmetrically expressed in activated satellite cells. ( a ) Immunostaining of satellite cells for MYOD (red), G-CSFR (green) and DAPI (blue) at day 5. Scale bar, 20 μm. ( b ) Immunostaining of satellite cells for G-CSFR (purple), PAX7 (green) and DAPI (blue) at day 3. Scale bar, 5 μm. ( c ) Immunostaining of dividing satellite cells on myofibres for G-CSFR (green), SDC4 (red) and DAPI (blue), as well as bright-field (BF) images, at 48 h (satellite cells with symmetric G-CSFR expression: n =51; satellite cells with asymmetric expression: n =3). Scale bar, 10 μm. ( d ) Immunostaining of dividing satellite cells on myofibres for G-CSFR (green), SDC4 (red) and DAPI (blue), as well as BF images, at 48 h. Scale bar, 10 μm. ( e , f ) Immunostaining of satellite cells on myofibres for SDC4 (red), G-CSFR (green) and DAPI (blue), as well as BF images, at 48 h. Scale bar, 10 μm. ( g ) Immunostaining of cultured dividing satellite cells for G-CSFR (purple), PAX7 (red), SDC4 (green) and DAPI (blue). Scale bar, 5 μm. ( h ) Immunostaining of cultured dividing satellite cells for G-CSFR (purple), PAX7 (red), MYOD (green) and DAPI (blue) at day 3 (among 273 dividing satellite cells, dividing satellite cells with symmetric G-CSFR expression: n =5; dividing satellite cells with asymmetric expression: n =268). Scale bar, 5 μm. All myofibres were obtained from ∼ 10-week-old wild-type mice. DAPI, 4',6-diamidino-2-phenylindole dihydrochloride. Full size image G-CSF increases SCs via the G-CSF–G-CSFR axis To elucidate whether G-CSFR signalling affects the populations of SCs, we examined the PAX7+ cell population in cultured myofibres from wild-type and G-CSFR-mutated ( csf3r −/− ) mice. At 0 and 24 h, there was no significant difference in the number of PAX7+ cells between wild-type and csf3r −/− mice; however, at 48 h, the csf3r−/− mice showed a significantly smaller number of PAX7+ cells than that of wild-type mice ( Fig. 3a,b ). At 24 h, most PAX7+ cells express MYOD, are activated and thereafter proliferate and commit to differentiation [21] , [22] , [23] . In the csf3r−/− mice, the number of MYOD+/PAX7+ cells was significantly decreased in PAX7+ cells activated for 24 h ( Fig. 3c,d ), suggesting that the genetic ablation of G-CSFR signalling negatively affects the population of activated SCs. We then examined the direct role of G-CSF on SCs from wild-type mice. At 72 h, the subpopulation of activated SCs had lost MYOD expression in vivo and on cultured myofibres [21] , [22] , [23] . Surprisingly, G-CSF significantly increased the population of SCs throughout the differentiation stages, including self-renewal SCs, as shown by the PAX7+/MYOD− cells at 72 h in wild-type mice; in addition, csf3r−/− mice showed significantly decreased numbers of SCs throughout the differentiation stages ( Fig. 3e,f ; Supplementary Table 1 ). To elucidate the effect of G-CSF on the population of PAX7+ cells in vivo , we examined SC behaviour in a cardiotoxin injury model ( Fig. 3g ). In the csf3r−/− mice, the population of PAX7+-expressing cells was significantly decreased at 14 days after cardiotoxin injection ( Fig. 3h,i ), suggesting that genetic G-CSFR signal ablation negatively affects the population of PAX7+ cells in vivo . 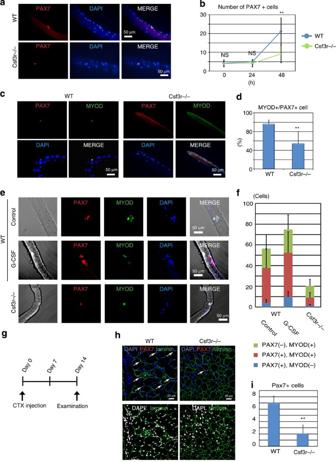Figure 3: G-CSF increases satellite cells in multiple differentiation stages. (a) Immunostaining of satellite cells on myofibres of∼10-week-old WT andcsf3r−/−mice for PAX7 (red) and DAPI (blue) at 48 h. Scale bar, 50 μm. (b) Time course of the number of satellite cells (PAX7+) at 0, 24 and 48 h per myofibre of WT andcsf3r−/−mice. Data are shown as mean±s.d. **P<0.01; equal variance Student’st-test. Each fibre number:n=20–29. (c) Immunostaining of satellite cells on myofibres of WT andcsf3r−/−mice for PAX7 (red), MYOD (green) and DAPI (blue) at 24 h. Scale bar, 50 μm. (d) The percentage of MYOD+/ PAX7+ satellite cells at 24 h. Data are shown as mean±s.d. **P<0.01; unequal variance Student’st-test. Each fibre number:n=29). (e) Immunostaining of satellite cells on myofibres of WT mice administered control and G-CSF andcsf3r −/−mice after being cultured for 72 h for PAX7 (red), MYOD (green) and DAPI (blue), as well as bright-field images. Scale bar, 50 μm. (f) Quantification of the number of PAX7−/MYOD+ (green), PAX7+/MYOD+ (red) or PAX7+/MYOD− (blue) satellite cells per myofibre. Data are shown as mean±s.d. One-way analysis of variance with Bonferroni'spost hoctest. Quantification information inSupplementary Table 1. (g) Time course of cardiotoxin (CTX) injection and examination for 8-week-old WT andcsf3r−/−mice. (h) Immunostaining of cross-sections of TA muscle of WT andcsf3r−/−mice at 14 days after CTX injection for laminin, PAX7 and DAPI. Upper panel: merged with laminin (green), PAX7 (red) and DAPI (blue). Lower panel: merged with laminin (green) and DAPI (white). Arrows indicate PAX7+/DAPI+ cells. Scale bar, 20 μm. (i) Number of PAX7+/DAPI+ cells per 100 myocytes of WT andcsf3r−/−mice. Data are shown as mean±s.d. **P<0.01; unequal variance Student’st-test.n=5–6 per group. DAPI, 4',6-diamidino-2-phenylindole dihydrochloride; WT, wild type. Figure 3: G-CSF increases satellite cells in multiple differentiation stages. ( a ) Immunostaining of satellite cells on myofibres of ∼ 10-week-old WT and csf3r−/− mice for PAX7 (red) and DAPI (blue) at 48 h. Scale bar, 50 μm. ( b ) Time course of the number of satellite cells (PAX7+) at 0, 24 and 48 h per myofibre of WT and csf3r−/− mice. Data are shown as mean±s.d. ** P <0.01; equal variance Student’s t -test. Each fibre number: n =20–29. ( c ) Immunostaining of satellite cells on myofibres of WT and csf3r−/− mice for PAX7 (red), MYOD (green) and DAPI (blue) at 24 h. Scale bar, 50 μm. ( d ) The percentage of MYOD+/ PAX7+ satellite cells at 24 h. Data are shown as mean±s.d. ** P <0.01; unequal variance Student’s t -test. Each fibre number: n =29). ( e ) Immunostaining of satellite cells on myofibres of WT mice administered control and G-CSF and csf3r −/− mice after being cultured for 72 h for PAX7 (red), MYOD (green) and DAPI (blue), as well as bright-field images. Scale bar, 50 μm. ( f ) Quantification of the number of PAX7−/MYOD+ (green), PAX7+/MYOD+ (red) or PAX7+/MYOD− (blue) satellite cells per myofibre. Data are shown as mean±s.d. One-way analysis of variance with Bonferroni's post hoc test. Quantification information in Supplementary Table 1 . ( g ) Time course of cardiotoxin (CTX) injection and examination for 8-week-old WT and csf3r−/− mice. ( h ) Immunostaining of cross-sections of TA muscle of WT and csf3r−/− mice at 14 days after CTX injection for laminin, PAX7 and DAPI. Upper panel: merged with laminin (green), PAX7 (red) and DAPI (blue). Lower panel: merged with laminin (green) and DAPI (white). Arrows indicate PAX7+/DAPI+ cells. Scale bar, 20 μm. ( i ) Number of PAX7+/DAPI+ cells per 100 myocytes of WT and csf3r−/− mice. Data are shown as mean±s.d. ** P <0.01; unequal variance Student’s t -test. n =5–6 per group. DAPI, 4',6-diamidino-2-phenylindole dihydrochloride; WT, wild type. Full size image We previously showed that G-CSF apparently activates JNK and p38 signalling in cultured myoblasts [9] . Therefore, we examined whether these pathways are active in activated SCs. Immunostaining for pJNK and pp38 revealed that both JNK and p38 are activated in G-CSFR+ SCs ( Fig. 4a ; Supplementary Fig. 3a ). The p38 pathway is required for SC activation and MYOD induction following proliferation [24] ; herein, p38 inhibition in single myofibres decreased the population of PAX7−/MYOD+ SCs with or without G-CSF ( Supplementary Fig. 3b,c ; Supplementary Table 1 ). Although JNK signalling is involved in myoblast differentiation [25] , its role in SC behaviour remains unclear. In paired PAX7+ cells, the G-CSFR-expressing daughter cells highly expressed activated JNK, whereas the other daughter cells without G-CSFR expression did not ( Fig. 4b ). JNK inhibition also strongly reduced the number of PAX7+/MYOD− and PAX7+/MYOD+ cells in single myofibres ( Fig. 4c,d ; Supplementary Table 1 ). These data indicated that G-CSF increases both activated and self-renewal SCs through the G-CSF–G-CSFR–JNK axis, suggesting that G-CSF could increase long-term regeneration in chronic skeletal muscle injury through maintenance of the SC pool. 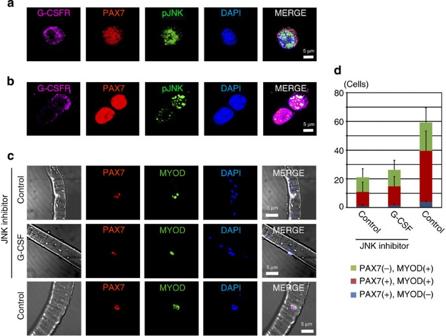Figure 4: G-CSF increases satellite cells through the G-CSF–G-CSFR–JNK axis. (a) Immunostaining of satellite cells for G-CSFR (purple), PAX7 (red), pJNK (green) and DAPI (blue) at day 3. Scale bar, 5 μm. (b) Immunostaining of dividing satellite cells for G-CSFR (purple), PAX7 (red), pJNK (green) and DAPI (blue) at day 3. Scale bar, 5 μm. (c) Immunostaining of satellite cells on myofibres of WT mice for PAX7 (red), MYOD (green) and DAPI (blue), as well as bright-field images, following JNK inhibitor administration with or without G-CSF at 72 h. Scale bar, 50 μm. (d) Quantification of the number of PAX7−/MYOD+ (green), PAX7+/MYOD+ (red) or PAX7+/MYOD− (blue) satellite cells per myofibre. Data are shown as mean±s.d. One-way analysis of variance with Bonferroni'spost hoctest. Quantification information inSupplementary Table 1. DAPI, 4',6-diamidino-2-phenylindole dihydrochloride. Figure 4: G-CSF increases satellite cells through the G-CSF–G-CSFR–JNK axis. ( a ) Immunostaining of satellite cells for G-CSFR (purple), PAX7 (red), pJNK (green) and DAPI (blue) at day 3. Scale bar, 5 μm. ( b ) Immunostaining of dividing satellite cells for G-CSFR (purple), PAX7 (red), pJNK (green) and DAPI (blue) at day 3. Scale bar, 5 μm. ( c ) Immunostaining of satellite cells on myofibres of WT mice for PAX7 (red), MYOD (green) and DAPI (blue), as well as bright-field images, following JNK inhibitor administration with or without G-CSF at 72 h. Scale bar, 50 μm. ( d ) Quantification of the number of PAX7−/MYOD+ (green), PAX7+/MYOD+ (red) or PAX7+/MYOD− (blue) satellite cells per myofibre. Data are shown as mean±s.d. One-way analysis of variance with Bonferroni's post hoc test. Quantification information in Supplementary Table 1 . DAPI, 4',6-diamidino-2-phenylindole dihydrochloride. Full size image G-CSF increases muscle regeneration in mdx mice Patients with DMD show progressive physical impairment leading to the death by 20–30 years of age, whereas a mouse model of DMD ( mdx mice) harbouring a dystrophin mutation has minimal physical impairment and a normal lifespan [26] . Indeed, mdx mice appear grossly normal ( Supplementary Fig. 4a ). However, pathological analysis revealed apparent muscle degeneration and regeneration in these mdx mice from 3 to 5 weeks of age ( Supplementary Fig. 4b ). Myocyte numbers in the tibialis anterior (TA) muscle were decreased at 3 weeks of age, but were thereafter recovered ( Supplementary Fig. 4c ). Generally, healthy myocytes have peripherally located nuclei, and regenerating and regenerated myocytes have central nuclei. The mdx mice myocytes showed central nuclei from 4 weeks of age and increased in number up to 12 weeks of age ( Supplementary Fig. 4d ). These data suggested initial injury to the muscle fibres with subsequent regeneration to an almost normal state in the mdx mice. The histological observation of TA muscle showed strong G-CSFR expression in regenerating myocytes ( Supplementary Fig. 4e ), implicating the possible role of G-CSF in the muscle regeneration process. We then examined whether G-CSF administration would improve skeletal muscle regeneration in mdx mice. We examined the gross appearance and functional differences following daily intraperitoneal (i.p.) G-CSF injections from 3 to 5 weeks of age ( Fig. 5a ). Immunostaining for laminin showed the typically fine cellular architecture of TA muscle ( Fig. 5b ). The number of myocytes with central nuclei significantly increased with G-CSF administration at 5 weeks of age ( Fig. 5c ). The BF-45 antibody recognizes myosin heavy chain present during embryonic and neonatal skeletal muscle development and in newly formed adult regenerating myocytes [27] . Immunostaining for BF-45 in 4-week-old mice treated with G-CSF revealed significantly increased numbers of regenerating myocytes ( Fig. 5d,e ). Measuring the individual cross-sectional area of the myocytes further revealed a significantly increased proportion of small myocytes, indicating a substantial amount of newly formed regenerated myocytes at 5 weeks of age ( Fig. 5f ). Given that muscle size is a predictive value for muscle function, the demonstrated increase in the TA muscle perimeter in G-CSF-treated mice at 5 weeks of age suggested enhanced muscle function recovery ( Fig. 5g ). G-CSF also significantly improved exercise capacity in the mice by 5 weeks of age based on in vivo exercise tolerance testing ( Fig. 5h ). In a pure muscle function test, ex vivo tetanic force measurements and specific force examinations showed significantly improved muscle tension in the treated mice at 5 weeks of age ( Fig. 5i,j ). 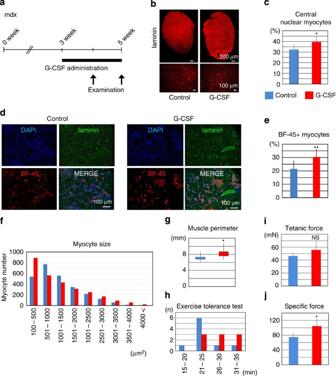Figure 5: G-CSF increases skeletal muscle regeneration inmdxmice. (a) Time course of G-CSF administration and examination inmdxmice. (b) Immunostaining of cross-sections of TA muscle for laminin at 5 weeks of agemdxmice. Scale bar, 200 μm (upper panel); 100 μm (lower panel). (c) The percentages of myocytes with central nuclei in cross-sections of TA muscle at 5 weeks of age. Data are shown as mean±s.d. *P<0.05; equal variance Student’st-test.n=8 per group. (d) Immunostaining of cross-sections of TA muscle for BF-45 (red), laminin (green) and DAPI (blue) at 4 weeks of age. Scale bar, 100 μm. (e) The percentages of BF-45-positive myocytes in cross-sections of TA muscle at 4 weeks of age. Data are shown as mean±s.d. **P<0.01; unequal variance Student’st-test.n=5 per group. (f) The individual fibre cross-sectional area of individual myocytes in cross-sections of TA muscles at 5 weeks of age. Data are shown as mean.n=6 per group. (g) Muscle perimeters of cross-sections of TA muscles at 5 weeks of age. Data are shown as box plot. Top, maximum; bottom, minimum. *P<0.05; equal variance Student’st-test.n=8 per group. (h) Exercise tolerance test results at 5 weeks of age.n=9 per group. (i) Tetanic force examination ofex vivoEDL muscle tension at 5 weeks of age. Data are shown as mean±s.d. No significant difference; unequal variance Student’st-test;n=6 per group. (j) Specific forces, which are the ratios of tetanic force to muscle size, measured at 5 weeks of age. Data are shown as mean±s.d. *P<0.05; unequal variance Student’st-test.n=5 per group. DAPI, 4',6-diamidino-2-phenylindole dihydrochloride; NS, not significant. Figure 5: G-CSF increases skeletal muscle regeneration in mdx mice. ( a ) Time course of G-CSF administration and examination in mdx mice. ( b ) Immunostaining of cross-sections of TA muscle for laminin at 5 weeks of age mdx mice. Scale bar, 200 μm (upper panel); 100 μm (lower panel). ( c ) The percentages of myocytes with central nuclei in cross-sections of TA muscle at 5 weeks of age. Data are shown as mean±s.d. * P <0.05; equal variance Student’s t -test. n =8 per group. ( d ) Immunostaining of cross-sections of TA muscle for BF-45 (red), laminin (green) and DAPI (blue) at 4 weeks of age. Scale bar, 100 μm. ( e ) The percentages of BF-45-positive myocytes in cross-sections of TA muscle at 4 weeks of age. Data are shown as mean±s.d. ** P <0.01; unequal variance Student’s t -test. n =5 per group. ( f ) The individual fibre cross-sectional area of individual myocytes in cross-sections of TA muscles at 5 weeks of age. Data are shown as mean. n =6 per group. ( g ) Muscle perimeters of cross-sections of TA muscles at 5 weeks of age. Data are shown as box plot. Top, maximum; bottom, minimum. * P <0.05; equal variance Student’s t -test. n =8 per group. ( h ) Exercise tolerance test results at 5 weeks of age. n =9 per group. ( i ) Tetanic force examination of ex vivo EDL muscle tension at 5 weeks of age. Data are shown as mean±s.d. No significant difference; unequal variance Student’s t -test; n =6 per group. ( j ) Specific forces, which are the ratios of tetanic force to muscle size, measured at 5 weeks of age. Data are shown as mean±s.d. * P <0.05; unequal variance Student’s t -test. n =5 per group. DAPI, 4',6-diamidino-2-phenylindole dihydrochloride; NS, not significant. Full size image Next, we examined whether G-CSF treatment would accelerate the regeneration process following cardiotoxin injury in mdx mice ( Fig. 6a ). The number of myocytes with central nuclei significantly increased by G-CSF administration in cardiotoxin-injured mdx mice ( Fig. 6b,c ). The number of BF-45+ myocytes was also significantly increased by G-CSF treatment ( Fig. 6d,e ). The TA muscle perimeter was also increased by G-CSF treatment in cardiotoxin-injured mdx mice ( Fig. 6f ). These data suggested that G-CSF significantly improves muscle function through myocyte regeneration in mdx mice. 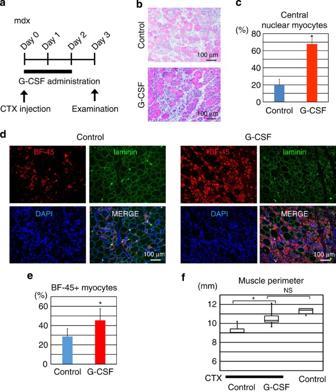Figure 6: G-CSF increases muscle regeneration inmdxmice after CTX injury. (a) Time course of CTX and G-CSF administration, and examination in 8-week-oldmdxmice. (b) Haematoxylin and eosin staining of cross-sections of TA muscle at day 3 after CTX injection. Scale bar, 100 μm. (c) The percentages of central nuclear myocytes in cross-sections of TA muscle at day 3 after CTX injection. Data are shown as mean±s.d. *P<0.05; unequal variance Student’st-test.n=4 per group. (d) Immunostaining of cross-sections of TA muscle for BF-45 (red), laminin (green) and DAPI (blue) at day 3 after CTX injection. Scale bar, 100 μm. (e) The percentages of BF-45-positive myocytes in cross-sections of TA muscle at day 3 after CTX injection. Data are shown as mean±s.d. *P<0.05; unequal variance Student’st-test.n=5 per group. (f) Muscle perimeters of cross-sections of TA muscle at day 3 after CTX injection. Data are shown as box plot. Top, maximum; bottom, minimum. *P<0.05; Student’st-test.n=4–6 per group. CTX, cardiotoxin; DAPI, 4',6-diamidino-2-phenylindole dihydrochloride; NS, not significant. Figure 6: G-CSF increases muscle regeneration in mdx mice after CTX injury. ( a ) Time course of CTX and G-CSF administration, and examination in 8-week-old mdx mice. ( b ) Haematoxylin and eosin staining of cross-sections of TA muscle at day 3 after CTX injection. Scale bar, 100 μm. ( c ) The percentages of central nuclear myocytes in cross-sections of TA muscle at day 3 after CTX injection. Data are shown as mean±s.d. * P <0.05; unequal variance Student’s t -test. n =4 per group. ( d ) Immunostaining of cross-sections of TA muscle for BF-45 (red), laminin (green) and DAPI (blue) at day 3 after CTX injection. Scale bar, 100 μm. ( e ) The percentages of BF-45-positive myocytes in cross-sections of TA muscle at day 3 after CTX injection. Data are shown as mean±s.d. * P <0.05; unequal variance Student’s t -test. n =5 per group. ( f ) Muscle perimeters of cross-sections of TA muscle at day 3 after CTX injection. Data are shown as box plot. Top, maximum; bottom, minimum. * P <0.05; Student’s t -test. n =4–6 per group. CTX, cardiotoxin; DAPI, 4',6-diamidino-2-phenylindole dihydrochloride; NS, not significant. Full size image Haploinsufficiency of G-CSFR induces lethality in mdx mice To clarify the roles of G-CSF in DMD, we next used csf3r −/− mice, which show a slight haematological disorder and a normal lifespan [28] , [29] . We hypothesized that breeding G-CSFR homozygote-knockout mdx mice ( mdx/csf3r −/− ) would produce mice with severely impaired muscle regeneration and function. Surprisingly, G-CSFR heterozygote mdx ( mdx/csf3r +/− ) mice showed early partial lethality after birth and late partial lethality at 3–5 weeks of age ( Fig. 7a ). These striking data indicated the importance of proper G-CSF signalling in DMD. The mdx , csf3r +/− and mdx/csf3r +/− mice were of normal gross appearance at post-natal day (P) P1 ( Fig. 7b ); however, mdx/csf3r +/− mice had significantly reduced body weights compared with mdx littermates ( Fig. 7c ). To elucidate the cause of early lethality, we examined the mice for gross appearance of the diaphragm and degenerative lesions by Evans blue staining. Lesions were largely absent from the mdx , csf3r +/− and wild-type mice, whereas the mdx/csf3r +/− mice showed obvious degenerative lesions ( Fig. 7d,e ). Diaphragm thickness was also significantly decreased in mdx/csf3r +/− mice compared with mdx littermates ( Fig. 7f ). The population of PAX7+ cells in diaphragm was also significantly decreased in mdx/csf3r +/− mice ( Fig. 7g,h ). Whole-body plethysmography indicated that mdx/csf3r +/− mice showed mildly impaired respiratory function ( Fig. 7i–k ). In addition, the surviving mdx/csf3r +/− mice showed consecutive body weight loss compared with csf3r +/− mice ( Fig. 7i ). Because most mdx/csf3r +/− mice with a strong phenotype died before 5 weeks of age and relative healthy mdx/csf3r +/− mice survive, the differences in body weight and respiratory function would be decreased thereafter. 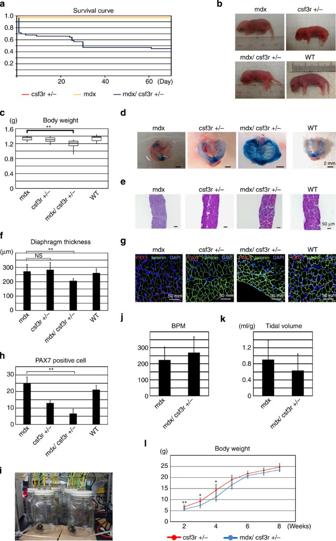Figure 7: G-CSF signalling is essential for the survival inmdxmice. (a) Kaplan–Meier survival curve ofcsf3r+/−(red,n=50),mdx(yellow,n=50) andmdx/csf3r+/−(blue,n=53) mice. (b) Gross appearance ofmdx,csf3r+/−,mdx/csf3r+/−and WT mice at post-natal day 1. (c) Body weights ofmdx(n=7),csf3r+/−(n=9),mdx/csf3r+/−(n=11) and WT (n=15) mice at post-natal day 1. Data are shown as box plot. Top, maximum; bottom, minimum. **P<0.01; unequal variance Student’st-test. (d) Evans blue staining of the diaphragm ofmdx,csf3r+/−,mdx/csf3r+/−and WT mice at post-natal day 1. (e) Haematoxylin and eosin staining of the diaphragm ofmdx,csf3r+/−,mdx/csf3r+/−and WT mice at post-natal day 1. Scale bar, 50 μm. (f) Diaphragm thickness ofmdx,csf3r+/−,mdx/csf3r+/−and WT mice at post-natal day 1 (n=5 per group). Data are shown as mean±s.d. **P<0.01; Student’st-test;n=5 per group. (g) Immunostaining of cross-sections of the diaphragm for PAX7 (red), laminin (green) and DAPI (blue) at post-natal day 1 ofmdx,csf3r+/−,mdx/csf3r+/−and WT mice. Scale bar, 50 μm. (h) Number of PAX7+/DAPI+ cells per 100 myocytes at post-natal day 1 ofmdx,csf3r+/−,mdx/csf3r+/−andWTmice. Data are shown as mean±s.d. **P<0.01; Student’st-test;n=5 per group. (i) Whole-body plethysmography to examine the respiratory function of individual mice. (j) Breath per min (BPM) in 8-week-oldmdxandmdx/csf3r+/−mice. Data are shown as mean±s.d. No significant difference; unequal variance Student’st-test;n=4 per group. (k) Tidal volume of 8-week-oldmdxandmdx/csf3r+/−mice. Data are shown as mean±s.d. No significant difference; unequal variance Student’st-test;n=4 per group. (l) Body weight growth curves ofcsf3r+/−andmdx/csf3r+/−mice from 2 to 8 weeks of age. Data are shown as mean±s.d. *P<0.05, **P<0.01; unequal variance Student’st-test;n=7 per group. DAPI, 4',6-diamidino-2-phenylindole dihydrochloride; NS, not significant; WT, wild type. Figure 7: G-CSF signalling is essential for the survival in mdx mice. ( a ) Kaplan–Meier survival curve of csf3r +/− (red, n =50), mdx (yellow, n =50) and mdx/csf3r +/− (blue, n =53) mice. ( b ) Gross appearance of mdx , csf3r +/− , mdx/csf3r +/− and WT mice at post-natal day 1. ( c ) Body weights of mdx ( n =7), csf3r +/− ( n =9), mdx/csf3r +/− ( n =11) and WT ( n =15) mice at post-natal day 1. Data are shown as box plot. Top, maximum; bottom, minimum. ** P <0.01; unequal variance Student’s t -test. ( d ) Evans blue staining of the diaphragm of mdx , csf3r +/− , mdx/csf3r +/− and WT mice at post-natal day 1. ( e ) Haematoxylin and eosin staining of the diaphragm of mdx , csf3r +/− , mdx/csf3r +/− and WT mice at post-natal day 1. Scale bar, 50 μm. ( f ) Diaphragm thickness of mdx , csf3r +/− , mdx/csf3r +/− and WT mice at post-natal day 1 ( n =5 per group). Data are shown as mean±s.d. ** P <0.01; Student’s t -test; n =5 per group. ( g ) Immunostaining of cross-sections of the diaphragm for PAX7 (red), laminin (green) and DAPI (blue) at post-natal day 1 of mdx , csf3r +/− , mdx/csf3r +/− and WT mice. Scale bar, 50 μm. ( h ) Number of PAX7+/DAPI+ cells per 100 myocytes at post-natal day 1 of mdx , csf3r +/− , mdx/csf3r +/− and WT mice. Data are shown as mean±s.d. ** P <0.01; Student’s t -test; n =5 per group. ( i ) Whole-body plethysmography to examine the respiratory function of individual mice. ( j ) Breath per min (BPM) in 8-week-old mdx and mdx/csf3r +/− mice. Data are shown as mean±s.d. No significant difference; unequal variance Student’s t -test; n =4 per group. ( k ) Tidal volume of 8-week-old mdx and mdx/csf3r +/− mice. Data are shown as mean±s.d. No significant difference; unequal variance Student’s t -test; n =4 per group. (l) Body weight growth curves of csf3r +/− and mdx/csf3r +/− mice from 2 to 8 weeks of age. Data are shown as mean±s.d. * P <0.05, ** P <0.01; unequal variance Student’s t -test; n =7 per group. DAPI, 4',6-diamidino-2-phenylindole dihydrochloride; NS, not significant; WT, wild type. Full size image In mdx mice, skeletal muscle degeneration and regeneration is prominent at 3–5 weeks of age. We therefore proposed that mdx/csf3r +/− mice might show deteriorating muscle regeneration and function around that age. Gross examination revealed a smaller body size in mdx/csf3r +/− and mdx/csf3r −/− mice at P7, and apparently smaller body size in mdx/csf3r −/− mice at P13 ( Fig. 8a ). Mdx/csf3r +/− mice that survived the initial early lethality prevalence showed significantly increased degeneration with decreased numbers of regenerating myocytes at ∼ 4 weeks of age that remained at ∼ 8 weeks of age ( Fig. 8b ). The myocyte number and TA muscle perimeter were also significantly decreased in mdx/csf3r +/− mice at 8 weeks of age ( Fig. 8c,d ). Ex vivo muscle tension examination also indicated significantly decreased tetanic and specific forces in the mdx/csf3r +/− mice compared with mdx mice ( Fig. 8e,f ). The population of PAX7+ cells was also significantly decreased in mdx/csf3r +/− mice ( Fig. 8g,h ). These results confirmed that G-CSF signal is crucial for skeletal muscle regeneration in mdx mice. 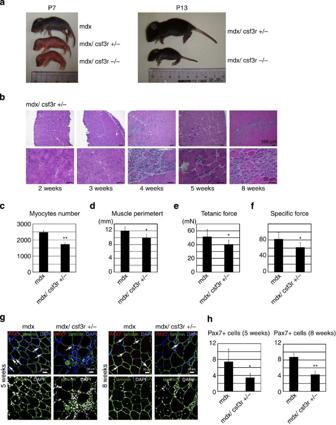Figure 8: Haploinsufficiency of G-CSFR reduces muscle regeneration inmdxmice. (a) Gross appearance analyses showing body size differences amongmdx,mdx/csf3r+/−andmdx/csf3r−/−mice at post-natal day 7 (left panel) and betweenmdx/csf3r+/−andmdx/csf3r−/−mice at post-natal day 13 (right panel). (b) Haematoxylin and eosin staining of cross-sections of TA muscle frommdx/csf3r+/−mice from 2 to 8 weeks of age are shown in the lower (upper panel) and higher (lower panel) magnified images. Scale bar, 100 μm (upper panel); 50 μm (lower panel). (c) The total numbers of myocytes in cross-sections of TA muscle at 8 weeks. Data are shown as mean±s.d. **P<0.01; unequal variance Student’st-test;n=5 per group. (d) Perimeters of cross-sections of TA muscle at 8 weeks of age. Data are shown as mean±s.d. *P<0.05; unequal variance Student’st-test;n=5 per group. (e) Tetanic force examination ofex vivoEDL muscle tension at 8 weeks of age. Data are shown as mean±s.d. *P<0.05; unequal variance Student’st-test;n=5 per group. (f) Specific forces, represented by tetanic force per muscle size ratios, at 8 weeks of age. Data are shown as mean±s.d. *P<0.05; unequal variance Student’st-test;n=6 per group. (g) Immunostaining of cross-sections of TA muscle frommdxandmdx/csf3r+/−mice at 5 and 8 weeks of age for laminin, PAX7 and DAPI. Upper panel: merged with laminin (green), PAX7 (red) and DAPI (blue). Lower panel: merged with laminin (green) and DAPI (white). Arrows indicate PAX7+/DAPI+ cells. Scale bar, 20 μm. (h) Number of PAX7+/DAPI+ cells per 100 myocytes ofmdxandmdx/csf3r+/−mice at 5 and 8 weeks of age. Data are shown as mean±s.d. *P<0.05, **P<0.01; unequal variance Student’st-test;n=5 per group. DAPI, 4',6-diamidino-2-phenylindole dihydrochloride; NS, not significant; WT, wild type. Figure 8: Haploinsufficiency of G-CSFR reduces muscle regeneration in mdx mice. ( a ) Gross appearance analyses showing body size differences among mdx , mdx/csf3r +/− and mdx/csf3r −/− mice at post-natal day 7 (left panel) and between mdx/csf3r +/− and mdx/csf3r −/− mice at post-natal day 13 (right panel). ( b ) Haematoxylin and eosin staining of cross-sections of TA muscle from mdx/csf3r +/− mice from 2 to 8 weeks of age are shown in the lower (upper panel) and higher (lower panel) magnified images. Scale bar, 100 μm (upper panel); 50 μm (lower panel). ( c ) The total numbers of myocytes in cross-sections of TA muscle at 8 weeks. Data are shown as mean±s.d. ** P <0.01; unequal variance Student’s t -test; n =5 per group. ( d ) Perimeters of cross-sections of TA muscle at 8 weeks of age. Data are shown as mean±s.d. * P <0.05; unequal variance Student’s t -test; n =5 per group. ( e ) Tetanic force examination of ex vivo EDL muscle tension at 8 weeks of age. Data are shown as mean±s.d. * P <0.05; unequal variance Student’s t -test; n =5 per group. ( f ) Specific forces, represented by tetanic force per muscle size ratios, at 8 weeks of age. Data are shown as mean±s.d. * P <0.05; unequal variance Student’s t -test; n =6 per group. ( g ) Immunostaining of cross-sections of TA muscle from mdx and mdx/csf3r +/− mice at 5 and 8 weeks of age for laminin, PAX7 and DAPI. Upper panel: merged with laminin (green), PAX7 (red) and DAPI (blue). Lower panel: merged with laminin (green) and DAPI (white). Arrows indicate PAX7+/DAPI+ cells. Scale bar, 20 μm. ( h ) Number of PAX7+/DAPI+ cells per 100 myocytes of mdx and mdx/csf3r +/− mice at 5 and 8 weeks of age. Data are shown as mean±s.d. * P <0.05, ** P <0.01; unequal variance Student’s t -test; n =5 per group. DAPI, 4',6-diamidino-2-phenylindole dihydrochloride; NS, not significant; WT, wild type. Full size image G-CSF supports the survival of severe DMD model mice The physically normal appearance of mdx mice could reflect a redundant function of the utrophin gene, a dystrophin paralogue. The mdx/utrn −/− mice that express neither dystrophin nor utrophin manifest severe dystrophy resembling human DMD [30] , [31] . These mice showed an apparently small body size compared with the mdx mice ( Supplementary Fig. 5a ), with prominent skeletal muscle degeneration that remained to a late stage of post-natal growth ( Supplementary Fig. 5b ). Total myocyte number in TA muscle was also decreased from 2 to 5 weeks of age in these mdx/utrn −/− mice, and recovered thereafter ( Supplementary Fig. 5c ), and central nuclear myocytes were apparent after 3 weeks ( Supplementary Fig. 5d ). G-CSFR was also expressed in regenerating myocytes in the mdx/utrn −/− mice ( Supplementary Fig. 5e ). To elucidate whether G-CSF improves skeletal muscle regeneration in these mice, we i.p. injected G-CSF using several schedules ( Fig. 9a ). After daily G-CSF injection from 3 to 5 weeks of age, muscle size was significantly increased in the G-CSF-treated animals at 5 weeks of age ( Fig. 9b,c ). G-CSF administration also significantly increased the moist muscle weight ratio of the gastrocnemius and quadriceps muscles in mdx/utrn −/− mice ( Fig. 9d ), as well as the numbers of regenerated myocytes and total myocytes in TA muscle ( Supplementary Fig. 6a,b ; Fig. 9g ). The number of BF-45+ myocytes was significantly increased by G-CSF treatment ( Fig. 9e,f ). The population of PAX7+ cell was also significantly increased by G-CSF treatment ( Supplementary Fig. 6c,d ). Ex vivo muscle functional analysis showed that tetanic and specific forces were significantly increased by G-CSF administration ( Fig. 9h,i ). These data suggested that G-CSF improves skeletal muscle regeneration and muscle function in mdx/utrn −/− mice. 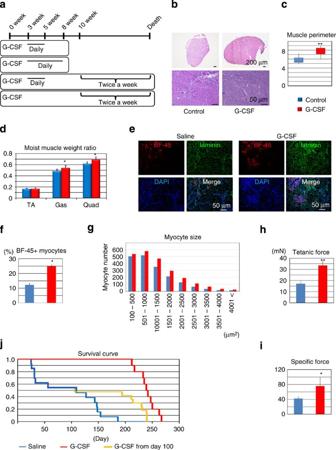Figure 9: G-CSF improves the survival of mice with severe muscular dystrophy. (a) Time course of G-CSF administration. (b) Haematoxylin and eosin staining of cross-sections of TA muscle frommdx/utrn−/−mice at 5 weeks of age (left: control; right: G-CSF administration). Scale bar, 200 μm (upper panel); 50 μm (lower panel). (c) Perimeters of cross-sections of TA muscle at 5 weeks of age. Data are shown as box plot. Top, maximum; bottom, minimum. **P<0.01; unequal variance Student’st-test;n=6 per group. (d) Ratios of moist muscle weight to body weight at 5 weeks of age. Data are shown as mean±s.d. *P<0.05; equal variance Student’st-test;n=9 per group. (e) Immunostaining of cross-sections of TA muscle for BF-45 (red), laminin (green) and DAPI (blue) at 4 weeks of age. Scale bar, 50 μm. (f) The percentages of BF-45-positive myocytes in cross-sections of TA muscle at 4 weeks of age. Data are shown as mean±s.d. **P<0.01; equal variance Student’st-test;n=5 per group. (g) The individual fibre cross-sectional areas of the myocytes in TA muscle at 5 weeks of age. Data are shown as mean;n=6 per group. (h) Tetanic force examination ofex vivoEDL muscle tension at 5 weeks of age is presented. Data are shown as mean±s.d. **P<0.01; unequal variance Student’st-test;n=5 per group. (i) Specific force results, represented by tetanic force per muscle size ratios. Data are shown as mean±s.d. *P<0.05; unequal variance Student’st-test;n=5 per group. (j) Kaplan–Meier survival curve ofmdx/utrn−/−mice without G-CSF (n=13), with G-CSF (n=10) or with G-CSF administration starting at day 100 (n=9). DAPI, 4',6-diamidino-2-phenylindole dihydrochloride. Figure 9: G-CSF improves the survival of mice with severe muscular dystrophy. ( a ) Time course of G-CSF administration. ( b ) Haematoxylin and eosin staining of cross-sections of TA muscle from mdx/utrn −/− mice at 5 weeks of age (left: control; right: G-CSF administration). Scale bar, 200 μm (upper panel); 50 μm (lower panel). ( c ) Perimeters of cross-sections of TA muscle at 5 weeks of age. Data are shown as box plot. Top, maximum; bottom, minimum. ** P <0.01; unequal variance Student’s t -test; n =6 per group. ( d ) Ratios of moist muscle weight to body weight at 5 weeks of age. Data are shown as mean±s.d. * P <0.05; equal variance Student’s t -test; n =9 per group. ( e ) Immunostaining of cross-sections of TA muscle for BF-45 (red), laminin (green) and DAPI (blue) at 4 weeks of age. Scale bar, 50 μm. ( f ) The percentages of BF-45-positive myocytes in cross-sections of TA muscle at 4 weeks of age. Data are shown as mean±s.d. ** P <0.01; equal variance Student’s t -test; n =5 per group. ( g ) The individual fibre cross-sectional areas of the myocytes in TA muscle at 5 weeks of age. Data are shown as mean; n =6 per group. ( h ) Tetanic force examination of ex vivo EDL muscle tension at 5 weeks of age is presented. Data are shown as mean±s.d. ** P <0.01; unequal variance Student’s t -test; n =5 per group. ( i ) Specific force results, represented by tetanic force per muscle size ratios. Data are shown as mean±s.d. * P <0.05; unequal variance Student’s t -test; n =5 per group. ( j ) Kaplan–Meier survival curve of mdx/utrn −/− mice without G-CSF ( n =13), with G-CSF ( n =10) or with G-CSF administration starting at day 100 ( n =9). DAPI, 4',6-diamidino-2-phenylindole dihydrochloride. Full size image The mdx/utrn −/− mice died at ∼ 3 to 5 weeks of age and after 100 days of age, resulting in 100% lethality by 180 days ( Fig. 9j , blue line). Finally, we showed that long-term G-CSF treatment could notably improve the survival of mdx/utrn −/− mice, with G-CSF injected daily from 3 to 5 weeks of age and twice a week after 10 weeks of age ( Fig. 9j , red line). It is clinically important to treat developed DMD; hence, the G-CSF was also injected from 10 weeks of age. G-CSF administration prolonged the survival of developed DMD model mice ( Fig. 9j , yellow line). Whole-body plethysmography then indicated that G-CSF administration significantly increased respiratory function, measured by tidal volume (TV), in the mdx/utrn −/− mice injected daily from 3 to 8 weeks of age ( Supplementary Fig. 6e ). The G-CSF-treated mdx/utrn −/− mice also showed improved physical activity at 150 days of age ( Supplementary Movie ). Although cardiomyopathy is one of the fatal phenotypes of DMD, heart morphology is not affected by G-CSF treatment ( Supplementary Fig. 6f,g ). These data strongly suggested that G-CSF improves skeletal muscle regeneration and function, and supports the survival of DMD model mice. Research over many years has sought to understand the mechanism of skeletal muscle stem cell behaviour and elucidate the precise pathogenesis underlying DMD and, in turn, to develop effective therapies. Although many promising therapeutic strategies have been developed in animal experiments [32] , most human clinical trials failed to show significant efficacy in patients with DMD [12] , [14] , [33] , [34] , [35] . In addition, with the exception of glucocorticoids, beneficial results with immunosuppressants were inconclusive [36] , [37] , [38] , [39] . Indeed, the precise mechanism by which glucocorticoids increase muscle strength in DMD is not known and its clinical effects are generally not sufficient. Improved or additional therapies for DMD are therefore urgently needed. G-CSF is a well-known cytokine that recruits hematopoietic cells [40] . The safety and side effects in humans were widely known from previously established clinical applications, which enable us to use G-CSF early in clinics. Our studies now highlight apparently encouraging the effects of G-CSF on DMD. In this work, we showed that G-CSFR is asymmetrically distributed in some activated SCs, and G-CSF successfully increases the population of SCs at the multi-differentiating stages. We successfully showed that G-CSF administration markedly improves the phenotype of DMD model mice. The quiescent state in SC is required for the long-term maintenance of skeletal muscle [41] . We showed that G-CSF increased the PAX7+/MYOD− self-renewal SCs. There are quiescent SCs among PAX7+/MYOD− SCs, but it remains unclear whether G-CSF would affect the quiescent SC population. Because G-CSFR is not expressed in PAX7+/MYOD− SCs, G-CSF signalling would not be directly involved in the transition from activated SCs to PAX7+/MYOD− SCs. Furthermore, it remains unclear how G-CSF signalling increases the population of PAX7+/MYOD− SCs. And intrinsic differences among heterogenic satellite stem cells are still unclear and a practical marker to distinguish the subpopulations of satellite stem cells is still missing. Further precise elucidation of molecular mechanisms may directly facilitate control of the quiescent SC pool. As a study limitation, we could not directly show that bone marrow cells would not be involved in the phenotype of DMD model. To determine whether bone marrow cells have a role in early lethality of haploinsufficiency for G-CSFR in the dystrophic background, we performed bone marrow transplantation using mdx/csf3r+/− mice of ∼ 3–4 weeks of age. There is no established method of bone marrow transplantation for pups earlier than those ages. We selected active eight mdx/csf3r+/− mice of ∼ 3–4 weeks of age and successfully performed bone marrow transplantation. One of eight mdx/csf3r + /− mice died at 3 weeks after wild-type bone marrow transplantation by 8 weeks of age, which is similar to the survival rate of active mdx/csf3r+/− mice without bone marrow transplantation. Although wild-type bone marrow cells could not rescue the lethality of mdx/csf3r + /− mice, bone marrow transplantation would preferably be performed in mdx/csf3r+/− mice 0 days of age; alternatively, skeletal muscle-specific G-CSFR-deficient mice would ideally be generated. We confirmed that the G-CSF/G-CSFR system is critically involved in muscle regeneration during the course of DMD in several mouse models. Given our findings, it is surprising that haploinsufficiency of G-CSFR leads to early lethality in mdx mice, indicating that dose reduction of the G-CSF/G-CSFR system cannot support the balance between degeneration and regeneration in these mouse models. We also showed that G-CSF administration markedly improves the phenotype of mdx/utrn −/− mice. Together, our data suggested that G-CSF could improve the phenotype of human DMD and could consequently form the basis of novel and effective therapies in the near future. Mice C57BL/6-background mdx mice were provided by Dr T. Sasaoka (Niigata University Niigata, Japan). The utrophin -knockout mice were a kind gift from Dr Kay E Davies (University of Oxford, Oxford, UK) [31] . The dystrophin–utrophin double-knockout male homozygous ( dystrophin −/ Y (mdx) , utrophin −/− ) mice were obtained by crossing those heterozygous ( mdx , utrophin +/− ) mice. The csf3r−/− mice were kindly gifted by Dr Daniel C. Link (Washington University School of Medicine, St Louis) [28] . Mice deficient in both dystrophin and csf3r were derived by the following breeding program: male csf3r -knockout ( csf3r−/− ) mice were mated with female C57B/6 m dx ( dystrophin −/X ) mice, resulting in all F1-generation mice being heterozygous for csf3r ( csf3r +/− ) and either heterozygous for the mdx mutation ( dystrophin −/X , females) or hemizygous for the mdx mutation ( dystrophin −/Y , males). All data were obtained from P1 to 20 weeks of age male mice. All experimental procedures and protocols were approved by the Animal Care and Use Committee of Keio University and conformed to the NIH Guidelines for the Care and Use of Laboratory Animals. Genotyping DNA was isolated from mouse tails using the Easy-DNA Kit (Invitrogen, CA, USA). PCR analysis to identify mutant dystrophin alleles used a forward primer complementary to mouse dystrophin (5′- CATAGTTATTAATGCATAGATATTCAG -3′) and reverse primers complementary to the wild-type allele (5′- GTCACTCAGATAGTTGAAGCCATTTAG -3′) or mouse mutant dystrophin allele (5′- GTCACTCAGATAGTTGAAGCCATTTAA -3′). PCR cycling conditions for both the reactions were as follows: 95 °C for 4 min; 34 cycles of 95 °C for 1 min, 55 °C for 1 min and 72 °C for 1 min, and 72 °C for 10 min. Each reaction yielded a 275-bp product. All PCR reactions were performed using the GoTaq DNA Polymerase kit (Promega, Madison, WI, USA). PCR analysis to assess the utrophin -knockout status used a forward primer complementary to exon 7 of mouse utrophin (5′- GTGAAGGATGTCATGAAAG -3′) and reverse primers complementary either to intron 7 (5′- TGAAGTCCGAAAGAGATACC -3′) or to the PGK promoter located within the Neo-knockout cassette (5′- ACGAGACTAGTGAGACGTGC -3′). PCR reactions were carried out under the following conditions: 35 cycles of 94 °C for 30 s, 57 °C for 30 s and 72 °C for 25 s. PCR analysis to determine mutant csf3r alleles used a forward primer complementary to mouse csf3r (5′- AGTTCACCAGGCAGGTGAGT -3′) and reverse primers complementary to wild-type alleles (5′- GTAGGCCTAGTTCATACCTG -3′) or mouse mutant csf3r alleles (5′- TCCAGACTGCCTTGGGAAAA -3′). The PCR cycling conditions for both reactions were as follows: 95 °C for 4 min, followed by 30 cycles of 95 °C for 30 sec, 60 °C for 30 sec and 72 °C for 45 sec. Each reaction yielded a 279-bp product for the wild-type allele and a 366-bp product for the mutant csf3r allele. All PCR reactions were conducted using the Taq DNA Polymerase kit (TaKaRa, Shiga, Japan). G-CSF treatment G-CSF (Neutrogin, 100 μg; Chugai, Tokyo, Japan) was diluted in 1 ml of saline (concentration of 100 μg ml −1 ). Short-term treatment for mdx mice involved daily i.p. injections of 5 μg G-CSF from 3 to 5 weeks of age using a 27-gauge needle. Middle-term treatment for mdx/utrn −/− mice involved daily i.p. injections from 3 to 8 weeks of age at 5 μg using a 27-gauge needle. Long-term treatment for mdx/utrn −/− mice involved daily i.p. injections from 3 to 5 weeks of age and twice weekly from 10 weeks of age at 5 μg using a 27-gauge needle. Late treatment for mdx/utrn −/− mice involved twice weekly i.p. injections from 10 weeks of age at 5 μg using a 27-gauge needle. Histological analysis Frozen section of TA muscle was stained by haematoxylin and eosin to measure the ratio of muscle regeneration. The fibre cross-sectional area was measured using software (BZ-H1C: Keyence, Osaka, Japan) from laminin-stained cross-sections of TA muscle. Micrographs were taken from each section at, × 10 and × 20 magnification with a digital camera (BIOREVO: Keyence). Evans blue (Sigma-Aldrich, MO, USA) was dissolved in PBS (0.15 M NaCl, 10 mM phosphate buffer, pH 7.0). Mice were i.p. injected with 0.5 ml 0.1% Evans blue at P1 using a 27-gauge needle and were killed 3 h later. Immunofluorescence All immunofluorescence was carried out on 6-μm-thick frozen sections, myofibres and SCs. The frozen sections were fixed with acetone (WAKO, Osaka, Japan) for 20 min at −30 °C. Myofibres and SCs were fixed with 4% paraformaldehyde for 20 min at room temperature. All samples were incubated with 0.1% Triton X-100 for 5 min at room temperature, washed and then incubated with the following primary antibodies: anti-G-CSF receptor (sc-9173, 1:50: Santa Cruz Biotechnology, CA, USA; sc-323898, 1:100, Santa Cruz Biotechnology), anti-laminin 2 (L0663, 1:1000, Sigma-Aldrich), anti-laminin (L9393, 1:1000, Sigma-Aldrich), anti-BF-45 (1:30, Developmental Studies Hybridoma Bank, IA, USA), anti-MyoD (sc-32758, 1:200, mouse; sc-304, 1:200, Santa Cruz Biotechnology), anti-Pax7 (sc-81648, 1:100, 1:40, Santa Cruz Biotechnology), anti-myogenin (ab1835, 1:100, Abcam, Camb, UK; sc-576 1:100, Santa Cruz Biotechnology), anti-syndecan-4 (ab24511, 1:100, Abcam), anti-phospho-SAPK/JNK (#9251 1:100, rabbit, Cell Signaling Technology, MA, USA) and anti-phospho-p38 (sc-7973, 1:100, mouse, Santa Cruz Biotechnology). After overnight incubation, bound antibodies were visualized with a secondary antibody conjugated with Alexa 488, Alexa 546 or Alexa 633 (Life Technologies, CA, USA). Nuclei were stained with 4',6-diamidino-2-phenylindole dihydrochloride (Life technologies). For Pax7 staining, an M.O.M. kit (Vector Laboratories) was used to block the endogenous mouse IgG. The images were recorded using a confocal laser microscope system (Carl Zeiss, Jena, Germany) and BIOREVO (Keyence). Muscle force measurements EDL muscles were isolated and removed from 5-week-old mice. The muscles were carefully mounted in a chamber filled with PBS (95% O 2 and 5% CO 2 ) and maintained at 30 °C. One tendon of the muscle was attached to a steel hook in the chamber, and the other was tied to the lever arm of a dual-mode servomotor system (Electronic Stimulator; NIHON KOHDEN, Tokyo, Japan) via 5-0 surgical silk. The muscles were stretched to the length at which a single twitch and tetanic force showed the highest amplitude (optimal length; L o ). The corresponding tetanic force was then measured at 150 Hz over 5-s intervals for a total of 20 min, with a rest period of 120 s to change the buffer. The muscles were adjusted to the optimum length ( L o ) before all force measurements. For comparative purposes, all force measurements were expressed per the total muscle unit cross-sectional area, which was calculated by dividing the muscle mass by the product of the length and the mammalian skeletal muscle density (1.056 mg mm −3 ). The specific force (N cm −2 ) was calculated with the muscle density assumed as 1.056 g cm −3 . Exercise tolerance tests Mice were subjected to an exhaustion treadmill test by placing them on the belt of a one-lane motorized treadmill (MK-680S Treadmill for Rats & Mice; Muromachi Kikai, Tokyo, Japan). The test was started at an incline of 0 at 5 m min −1 for 5 min; thereafter, the speed was increased by 1 m min −1 every minute. The end point of the test was when the mouse remained on the shocker plate for >20 s. Whole-body plethysmography Animals were placed in a free-moving chamber that was connected to a high-gain differential pressure transducer (Valydine MP45, Validyne, North Ridge, CA, USA). As the animal breathed, changes in the pressure were converted to signals representing the TV; these signals were amplified (BMA 830; CWE, Ardmore, PA, USA), recorded on a strip-chart recorder (Dash 10; Astro-Med, West Warwick, RI, USA) and stored in a computer with respiratory acquisition software for analysis. O 2 consumption and CO 2 production were measured by the open-circuit method using Beckman OM-14 and LB-2 analysers. The parameter TV was analysed in real time, then average values were calculated five times every 2 min for each serial 3-h period. The TV was normalized by dividing by the body weight. Myofibre isolation and culture Single myofibres were isolated from EDL muscles and digested in DMEM GltaMax (Gibco, CA, USA) with 0.2% type 1 collagenase at 37 °C for 90 min. Fibres were liberated by trituration in DMEM medium with Pasteur pipettes. Isolated myofibres were cultured in suspension in serum-coated dishes. The fibre medium contained 20% foetal bovine serum (Sigma-Aldrich), 1% chick embryo extract (US Biological, MA, USA) 1% penicillin–streptomycin (Gibco), and DMEM GltaMax (Gibco). Single myofibres were incubated at 37 °C with 5% CO 2 for the indicated times. For the treatments, G-CSF (Neutrogin; Chugai) was added to the fibre medium to a concentration of 0.375 ng ml −1 , p38 inhibitor (SB203580, CST) was added to the fibre medium at a concentration of 10 μM and JNK inhibitor (SP600125, Cell Signaling Technology) was added to the fibre medium at a concentration of 5 μM. Isolation of SCs We obtained SCs using single myofibre culture, during which the SCs began to migrate on Matrigel (BD Biosciences, CA, USA)-coated dishes. Single SCs were then placed in Matrigel-coated glass-base dishes (Asahi Glass, Tokyo, Japan) and were maintained in fibre medium at 37 °C with 5% CO 2 for 3 days to allow SCs to migrate off the fibre and onto the Matrigel-coated dishes. Statistical analysis Values are reported as the means±s.d. The data were analysed using StatView J-4.5 software. Comparisons between the two groups were performed with Student’s t -test. Comparisons among the groups were performed by one-way analysis of variance with Bonferroni's post hoc test. Scheffe’s F -test was used to determine the level of significance. The probability level accepted for significance was * P <0.05, ** P <0.01. How to cite this article: Hayashiji, N. et al . G-CSF supports long-term muscle regeneration in mouse models of muscular dystrophy. Nat. Commun. 6:6745 doi: 10.1038/ncomms7745 (2015).